Far-red light photoactivatable near-infrared fluorescent proteins engineered from a bacterial phytochrome The ability to modulate the fluorescence of optical probes can be used to enhance signal-to-noise ratios for imaging within highly autofluorescent environments, such as intact tissues and living organisms. Here, we report two bacteriophytochrome-based photoactivatable near-infrared fluorescent proteins, named PAiRFP1 and PAiRFP2. PAiRFPs utilize haem-derived biliverdin, ubiquitous in mammalian tissues, as the chromophore. Initially weakly fluorescent PAiRFPs undergo photoconversion into a highly fluorescent state with excitation/emission at 690/717 nm following a brief irradiation with far-red light. After photoactivation, PAiRFPs slowly revert back to initial state, enabling multiple photoactivation-relaxation cycles. Low-temperature optical spectroscopy reveals several intermediates involved in PAiRFP photocycles, which all differ from that of the bacteriophytochrome precursor. PAiRFPs can be photoactivated in a spatially selective manner in mouse tissues, and optical modulation of their fluorescence allows for substantial contrast enhancement, making PAiRFPs advantageous over permanently fluorescent probes for in vivo imaging conditions of high autofluorescence and low signal levels. Bacterial phytochrome photoreceptors (BphPs) are natural red/far-red water-soluble photoreceptors that belong to the phytochrome superfamily, which also includes photoreceptors from plants, fungi and cyanobacteria [1] , [2] , [3] . Phytochromes share common domain architecture, which consists of a photosensory core domain (PCD) and an output effector module usually represented by histidine kinase. In turn, PCD is formed by three distinct domains, PAS (Per-ARNT-Sim), GAF (cGMP phosphodiesterase/adenylate cyclase/FhlA transcriptional activator) and PHY (phytochrome-specific), connected with α-helix linkers [4] , [5] , [6] . All chromophore–protein interactions occur in the PCD, which is mainly responsible for the spectral and photochemical properties of phytochromes. A light-sensing moiety in all phytochromes is composed of linear tetrapyrrole bilins [2] . Specifically, BphPs utilize biliverdin IXα (BV) as a chromophore, which is the product of oxidation of haem by haem oxygenase [7] . BphP apoprotein autocatalytically and covalently attaches BV via a thioester bond to a cysteine side chain at the N -terminus of the PAS domain [2] , [8] . BphPs are reversibly photoconverted between two stable states, termed Pr and Pfr, respectively by ‘red’ (peaked at 680–710 nm) and ‘far-red’ (peaked at 740–760 nm) light. Upon absorbance of ‘red’ light, the Pr state photoconverts into the Pfr state and vice versa, whereas illumination of the Pfr state with ‘far-red’ light results in the appearance of the Pr state. Once generated by light illumination, the photoconverted Pr and Pfr states revert back into their respective ground states either relatively slowly and non-photochemically, by means of the process called dark reversion, or rapidly, upon illumination with ‘far-red’/‘red’ light [3] , [4] , [5] . BphPs adopting the Pfr ground state are called bathy BphPs [9] , [10] , [11] . The photoconversion of phytochromes is a multistep process typically consisting of an initial photoreaction followed by a number of the dark relaxation steps [12] , [13] . The photoinduced Pr→Pfr and Pfr→Pr conversions were shown to proceed via distinct pathways involving different metastable intermediates (see reviews for details [4] , [5] ). The first intermediates formed after Pr and Pfr photoconversion are ascribed as lumi-R and lumi-F, respectively [14] . These photoproducts further undergo dark relaxation into intermediates designated by the prefix meta. For instance, meta-Ra and meta-Rb are relaxations of lumi-R, whereas meta-Fa and meta-Fb are relaxations of lumi-F ( Supplementary Fig. S1 ) (ref. 14 ). Intermediates differ from each other in their absorption spectra and can be stabilized at certain low temperatures in water buffers [15] , [16] , [17] , [18] , [19] . Compared with genetically encoded probes of blue, green or red fluorescent colors, near-infrared (NIR) fluorescent proteins (FPs) are superior for deep-tissue and whole-body imaging of small mammals [20] , [21] . This is because of low tissue autofluorescence and light scattering and minimal absorbance of melanin, water and haemoglobin in the NIR spectral region of ~650–900 nm, which is termed the NIR ‘optical window’ of mammalian tissue [22] . BphPs possess properties that make them potential templates for engineering NIR FPs. Firstly, BphPs can be readily expressed in mammalian cells and tissues, requiring no enzymes or exogenous cofactors [20] , [21] , [23] . Secondly, BphPs exhibit absorbance and fluorescence spectra, which lie within the NIR ‘optical window’ and are red-shifted relative to other types of phytochromes [3] and their fluorescent derivatives [24] , [25] , [26] . Recently, the PAS-GAF domains of several BphPs have been developed into NIR FPs, such as IFP1.4 and iRFP, and applied to whole-body imaging [20] , [21] , [23] . To further extend this set of genetically coded fluorescent tools for imaging in NIR ‘optical window’, we designed photoactivatable (PA) NIR FPs using one of the recently proposed strategies of BphP-based NIR FP engineering [27] . The capability to control spectral properties of PA FPs with light of a specific wavelength and intensity allows for optical labelling and tracking of proteins, organelles and living cells in a spatiotemporal manner, which is not possible with conventional FPs [28] . In addition, PA FPs can improve the achievable signal-to-background ratio, thus allowing higher resolution in samples containing substantial autofluorescence backgrounds [29] . In this paper, we apply molecular evolution to a bathy BphP from Agrobacterium tumefaciens C58 , called At BphP2 (refs 8 , 10 , 30 , 31 ), and develop two PA NIR FPs, named PAiRFP1 and PAiRFP2. We then study PAiRFP photoconversion mechanisms using a low-temperature ultraviolet-visible spectroscopy. Furthermore, we utilize PAiRFPs for in vivo fluorescence imaging and demonstrate spatially selective photoactivation of PAiRFPs in small regions of tumours in living mice. Lastly, an optical modulation of PAiRFPs fluorescent states allows us to substantially enhance the imaging contrast in early-stage tumours in vivo , resulting in the signal-to-background ratio values several-fold higher than for permanently fluorescent iRFP. Development of PAiRFPs We found that the Pfr state of At BphP2 protein truncated following PCD (termed AtPCD, amino acids 1–502 of At BphP2) can be photoconverted into the Pr state using both 660 and 750 nm light. Similar results were reported for the full-length At BphP2 protein [10] , [32] . However, the Pr state of the AtPCD protein is unstable and undergoes rapid dark reversion into Pfr with a half-time of 11 s ( Supplementary Fig. S2 ) (ref. 33 ). To stabilize the Pr state and enhance its fluorescence without interfering the Pfr→Pr photoconversion, a gene encoding AtPCD was subjected to several rounds of directed molecular evolution. Each round started from generation of library of mutants using random mutagenesis. The obtained library was co-expressed with haem oxygenase in Escherichia coli and screened using fluorescence-activated cell sorting (FACS), followed by selection of the appropriate clones on petri dishes using a fluorescence stereomicroscope equipped with 660 and 750 nm light-emitting diode (LED) arrays. After the first round, we have identified a weakly PA mutant, called At/660-I#1, having five substitutions compared with AtPCD. The At/660-I#1 mutant, initially in the non-fluorescent Pfr state, underwent almost complete photoconversion into the Pr state under both 660 and 750 nm illumination and after photoconversion reverted back into the initial state with a half-time of 4.1 min ( Supplementary Table S1 and Supplementary Fig. S3 ). Consequently, At/660-I#1 was used as a template for random mutagenesis, aimed to select PA NIR FPs with increased photoactivation contrast, enhanced brightness, blocked Pr→Pfr photoconversion and slowed or disabled dark reversion. In the subsequent rounds of molecular evolution, we used 660 nm photoactivation light as opposed to 750 nm light, for screening of PA NIR FP desirable variants. Light at 660 nm was advantageous because of the wide availability of light sources emitting at 700 nm and shorter wavelengths such as LEDs and arc lamp sources. The latter are often equipped with 700 nm cut-off filters in a light path that blocks light at 750 nm. In addition, high-power 660 nm light could be used to select clones that do not exhibit Pr→Pfr photoconversion under exposure to ~660 nm lower power probing light, which is used to excite fluorescence of the Pr state. As a result, we found two variants with slightly different phenotypes, designated PAiRFP1 and PAiRFP2. PAiRFP1 exhibited higher photoactivation contrast than PAiRFP2, but fourfold faster dark reversion. To understand an effect of the introduced mutations, we characterized spectral and biochemical properties of several mutants found during the molecular evolution of the AtPCD protein ( Supplementary Table S1 , Supplementary Figs S4 and S5 ). The introduced mutations mainly resulted in the increase of brightness and photoactivation contrast and in the decrease of dark reversion rates. Characterization of purified PAiRFPs We further compared properties of PAiRFP1 and PAiRFP2 with those of the AtPCD template and common permanently fluorescent iRFP [20] . Both PAiRFPs could exist in two stable interconvertable states, which we denoted as the relaxed and photoactivated states. 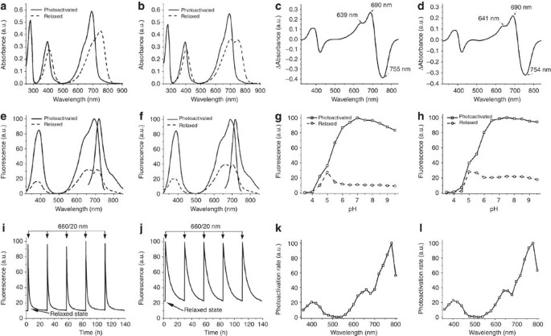Figure 1: Spectral and biochemical properties of PAiRFP1 and PAiRFP2in vitro. Absorbance spectra of the relaxed (dashed line) and photoactivated (solid line) PAiRFP1 (a) and PAiRFP2 (b). Difference spectra ‘relaxed’ minus ‘photoactivated’ for PAiRFP1 (c) and PAiRFP2 (d). Fluorescence spectra of the relaxed (dashed line) and photoactivated (solid line) PAiRFP1 (e) and PAiRFP2 (f). Equilibrium pH dependence for fluorescence of the relaxed (circles) and photoactivated (squares) PAiRFP1 (g) and PAiRFP2 (h). Fluorescence of the relaxed form was normalized to the maximal fluorescence of the photoactivated form. Time courses of the PAiRFP1 (i) and PAiRFP2 (j) fluorescence during multiple cycles of photoactivation and subsequent relaxation in the dark. After purification, the protein was briefly photoactivated with 660 nm light (26 mW cm−2). After the protein reached the relaxed state in the dark, it was briefly photoactivated again with 660 nm light (26 mW cm−2). Fluorescence in the photoactivated state was normalized to 100%. Spectral dependence of the maximal photoactivation rate for PAiRFP1 (k) and PAiRFP2 (l). The maximal values of the photoactivation rates were normalized to the light power in each wavelength band. Characteristics of PAiRFP1 and PAiRFP are summarized in Table 1 and Fig. 1 . The difference absorbance spectra for PAiRFPs demonstrated the characteristic phytochrome signature [8] , [33] , [34] , [35] , with maxima at ~690 and ~755 nm for the Pr and Pfr forms, respectively ( Fig. 1c ), similar to those of parental AtPCD [33] ( Supplementary Fig. S6 ). After photoactivation, both PAiRFPs slowly reverted back to the relaxed state with the half-times of 58 and 233 min, respectively, enabling multiple photoactivation-relaxation cycles without substantial changes in fluorescence brightness, relaxation rates, and photoactivation contrast ( Fig. 1i ). Table 1 Spectral and photochemical characteristics of PAiRFPs in comparison with AtPCD and iRFP. Full size table Figure 1: Spectral and biochemical properties of PAiRFP1 and PAiRFP2 in vitro . Absorbance spectra of the relaxed (dashed line) and photoactivated (solid line) PAiRFP1 ( a ) and PAiRFP2 ( b ). Difference spectra ‘relaxed’ minus ‘photoactivated’ for PAiRFP1 ( c ) and PAiRFP2 ( d ). Fluorescence spectra of the relaxed (dashed line) and photoactivated (solid line) PAiRFP1 ( e ) and PAiRFP2 ( f ). Equilibrium pH dependence for fluorescence of the relaxed (circles) and photoactivated (squares) PAiRFP1 ( g ) and PAiRFP2 ( h ). Fluorescence of the relaxed form was normalized to the maximal fluorescence of the photoactivated form. Time courses of the PAiRFP1 ( i ) and PAiRFP2 ( j ) fluorescence during multiple cycles of photoactivation and subsequent relaxation in the dark. After purification, the protein was briefly photoactivated with 660 nm light (26 mW cm −2 ). After the protein reached the relaxed state in the dark, it was briefly photoactivated again with 660 nm light (26 mW cm −2 ). Fluorescence in the photoactivated state was normalized to 100%. Spectral dependence of the maximal photoactivation rate for PAiRFP1 ( k ) and PAiRFP2 ( l ). The maximal values of the photoactivation rates were normalized to the light power in each wavelength band. Full size image Next, photoactivation properties of PAiRFPs were studied in more detail. Both PAiRFPs had a similar spectral dependence of the photoactivation rates, with maximal efficiencies of photoactivation observed at 780 nm ( Fig. 1k ). To estimate minimal light intensities required for complete photoactivation of PAiRFPs, we used 660 nm light from 0.012 to 26 mW cm −2 . The complete photoactivation of both PAiRFPs was achieved at the light power of ~2 mW cm −2 . Photoactivation of PAiRFPs at low temperature We used low-temperature ultraviolet-visible spectroscopy to study PAiRFP photoconversion photoproducts, and dark relaxation intermediates photoconversion under 660 and 750 nm light irradiation. After complete relaxation, PAiRFP proteins were flash frozen in liquid nitrogen and subsequently irradiated with 660 or 750 nm light. After the brief irradiation (about 10 s), the absorption spectra displayed significant changes, which possibly indicated accumulation of the intermediate states ( Fig. 2a ). PAiRFP1 absorbance spectra recorded after 660 or 750 nm illumination had slightly different profiles and exhibited maxima at 693 and 704 nm ( Fig. 2a ). The difference PAiRFP1 spectra indicated formation of at least two overlapping absorption bands in the ‘red’ region ( Fig. 2b ). For PAiRFP2, illumination with 660 or 750 nm light yielded very similar absorbance spectra peaked at 700 nm, with the only difference in the ‘red’ shoulder of the 660 nm illuminated sample ( Fig. 2c ). In the ‘red’ region, the difference PAiRFP2 spectra consisted of at least two overlapping absorption bands as well, with maxima around 630 and 700 nm. Under the same conditions, AtPCD also demonstrated substantial changes in absorbance spectra ( Supplementary Fig. S8 ). It should be noted that the absorbance bands of phytochromes usually shift to longer wavelength upon decreasing the temperature [16] , [17] . 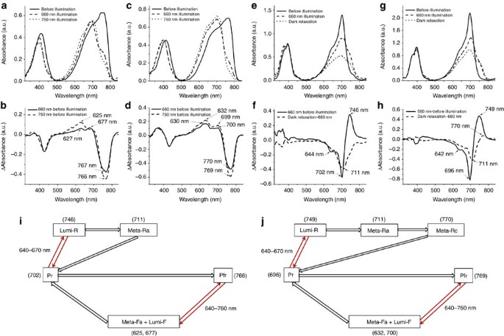Figure 2: Spectroscopy of intermediate products of PAiRFP1 and PAiRFP2 photoconversion. (a) Absorbance spectra of relaxed PAiRFP1 measured at 77 K before illumination (solid line), after 10 s of 660 nm illumination (dashed line) and after 10 s of 750 nm illumination (dotted line). (b) Difference spectra for phototransformation of relaxed PAiRFP1 at 77 K: ‘660 nm illumination’ minus ‘before illumination’ (solid line), and ‘750 nm illumination’ minus ‘before illumination’ (dashed line). (c) Absorbance spectra of relaxed PAiRFP2 measured at 77 K before illumination (solid line), after 10 s of 660 nm illumination (dashed line) and after 10 s of 750 nm illumination (dotted line). (d) Difference spectra for phototransformation of relaxed PAiRFP2 at 77 K: ‘660 nm illumination’ minus ‘before illumination’ (solid line), and ‘750 nm illumination’ minus ‘before illumination’ (dashed line). (e) Absorbance spectra of photoactivated PAiRFP1 measured before illumination at 77 K (solid line), and after 10 s of 660 nm illumination at 77 K (dashed line) and subsequent dark relaxation at 245 K (dotted line). (f) Difference spectra for phototransformation of photoactivated PAiRFP1 at low temperature: ‘660 nm illumination’ minus ‘before illumination’ (solid line), and ‘dark relaxation’ minus ‘660 nm illumination’ (dashed line). (g) Absorbance spectra of photoactivated PAiRFP2 measured before illumination at 77 K (solid line), and after 10 s of 660 nm illumination at 77 K (dashed line) and subsequent dark relaxation at 245 K (dotted line). (h) Difference spectra for phototransformation of photoactivated PAiRFP2 at low temperature: ‘660 nm illumination’ minus ‘before illumination’ (solid line) and ‘dark relaxation’ minus ‘660 nm illumination’ (dashed line). (i,j) Schematic representation of the proposed photocylces for PAiRFP1 (i) and PAiRFP2 (j). Values in the brackets denote wavelength of difference spectrum peaks. The indicated absorbance maxima of the intermediates, measured at low temperatures, can be different at room temperature where they likely will shift by 10–15 nm to shorter wavelengths, as was observed for wild-type phytochromes.16,17Arrows indicate photoreaction (thin red) or dark relaxation (wide black). Figure 2: Spectroscopy of intermediate products of PAiRFP1 and PAiRFP2 photoconversion. ( a ) Absorbance spectra of relaxed PAiRFP1 measured at 77 K before illumination (solid line), after 10 s of 660 nm illumination (dashed line) and after 10 s of 750 nm illumination (dotted line). ( b ) Difference spectra for phototransformation of relaxed PAiRFP1 at 77 K: ‘660 nm illumination’ minus ‘before illumination’ (solid line), and ‘750 nm illumination’ minus ‘before illumination’ (dashed line). ( c ) Absorbance spectra of relaxed PAiRFP2 measured at 77 K before illumination (solid line), after 10 s of 660 nm illumination (dashed line) and after 10 s of 750 nm illumination (dotted line). ( d ) Difference spectra for phototransformation of relaxed PAiRFP2 at 77 K: ‘660 nm illumination’ minus ‘before illumination’ (solid line), and ‘750 nm illumination’ minus ‘before illumination’ (dashed line). ( e ) Absorbance spectra of photoactivated PAiRFP1 measured before illumination at 77 K (solid line), and after 10 s of 660 nm illumination at 77 K (dashed line) and subsequent dark relaxation at 245 K (dotted line). ( f ) Difference spectra for phototransformation of photoactivated PAiRFP1 at low temperature: ‘660 nm illumination’ minus ‘before illumination’ (solid line), and ‘dark relaxation’ minus ‘660 nm illumination’ (dashed line). ( g ) Absorbance spectra of photoactivated PAiRFP2 measured before illumination at 77 K (solid line), and after 10 s of 660 nm illumination at 77 K (dashed line) and subsequent dark relaxation at 245 K (dotted line). ( h ) Difference spectra for phototransformation of photoactivated PAiRFP2 at low temperature: ‘660 nm illumination’ minus ‘before illumination’ (solid line) and ‘dark relaxation’ minus ‘660 nm illumination’ (dashed line). ( i , j ) Schematic representation of the proposed photocylces for PAiRFP1 ( i ) and PAiRFP2 ( j ). Values in the brackets denote wavelength of difference spectrum peaks. The indicated absorbance maxima of the intermediates, measured at low temperatures, can be different at room temperature where they likely will shift by 10–15 nm to shorter wavelengths, as was observed for wild-type phytochromes. [16] , [17] Arrows indicate photoreaction (thin red) or dark relaxation (wide black). Full size image It has been shown that illumination of the Pr state of the wild-type phytochromes at temperatures <170 K results in the formation of the lumi-R photoproduct, which can further undergo dark relaxation into the meta-Ra and meta-Rc intermediates [12] , [13] , [14] , [16] . Indeed, after brief 660 nm irradiation of flash-frozen photoactivated PAiRFPs at 77 K, we observed formation of a pronounced shoulder at ~746–749 nm, which could be ascribed to the lumi-R state ( Fig. 2e-h ). The subsequent dark relaxation of 660 nm illuminated samples at 245 K resulted in a noticeable decrease of this absorbance band ( Fig. 2e ), which, upon thawing, completely reverted back into the band corresponding to photoactivated PAiRFPs. Overall, these spectroscopic data suggest the following photocycles for PAiRFPs ( Fig. 2i ) (see also Supplementary Note 1 ). Behaviour of PAiRFPs in cultured cells To characterize PAiRFPs in mammalian cells, we transiently transfected HeLa cells with plasmids encoding non-targeted PAiRFPs. The cells also co-expressed enhanced green fluorescent protein (EGFP) for the purpose of normalizing transfection efficiency. No exogenous haem oxygenase was co-expressed. The cells were analysed using epifluorescence microscopy and flow cytometry ( Fig. 3 ). 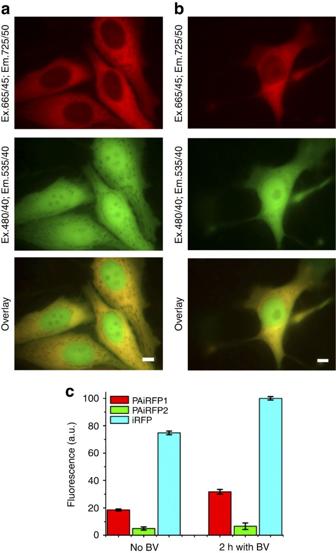Figure 3: Properties of PAiRFP1 and PAiRFP2 in cultured mammalian cells. Fluorescence images of transiently transfected HeLa cells co-expressing PAiRFP1 (a) and PAiRFP2 (b) with EGFP. Scale bar, 10 μm. (c) Mean NIR fluorescence intensity of the double-positive, transiently transfected HeLa cells normalized to transfection efficiency (EGFP signal), absorbance of the respective protein at 640 nm and overlap of the fluorescence spectrum of the respective protein with the transmission of the emission filter. NIR fluorescence intensities were analysed using flow cytometer with 640 nm excitation laser. Error bars, s.d. (n=3). Figure 3: Properties of PAiRFP1 and PAiRFP2 in cultured mammalian cells. Fluorescence images of transiently transfected HeLa cells co-expressing PAiRFP1 ( a ) and PAiRFP2 ( b ) with EGFP. Scale bar, 10 μm. ( c ) Mean NIR fluorescence intensity of the double-positive, transiently transfected HeLa cells normalized to transfection efficiency (EGFP signal), absorbance of the respective protein at 640 nm and overlap of the fluorescence spectrum of the respective protein with the transmission of the emission filter. NIR fluorescence intensities were analysed using flow cytometer with 640 nm excitation laser. Error bars, s.d. ( n= 3). Full size image Fluorescence signal of PAiRFPs was evenly distributed within the cytosol of living HeLa cells without aggregation or nonspecific localization ( Fig. 3a ). The PAiRFP proteins were excluded from the nucleus possibly because of the size (56.6 kDa × 2 for a dimer). The effective brightness of PAiRFP1 and PAiRFP2 in cells was 25% and 7% relative to iRFP, respectively. Treatment with 25 μM of exogenous BV for 2 h increased the brightness of PAiRFP1 cells by 1.7-fold and PAiRFP2 and iRFP cells by 1.3-fold ( Fig. 2c ). Photobleaching half-times for PAiRFP1 and PAiRFP2 in cells were 2.9 and 3.9 min, respectively ( Table 1 ). Both PAiRFPs demonstrated irreversible photobleaching under arc lamp illumination on a wide-field microscope ( Supplementary Fig. S9 ). Based on these photobleaching curves, there is no photochromism (that is, reversible phototransformation between two states with distinct spectral properties) for either PAiRFP. Imaging of PAiRFPs in live mice To examine applicability of PAiRFPs for in vivo imaging, we used a xenograft mouse model. Preclonal mixtures of rat adenocarcinoma MTLn3 cells stably expressing PAiRFPs were injected into the mammary glands of immunocompromised mice. MTLn3 cells expressing iRFP were injected into separate animals as a control. After cell transplantation, mammary tumours were allowed to grow over a 4-week period and imaged using an IVIS Spectrum instrument. Fluorescence signals of both photoactivated PAiRFPs and iRFP were first detected 1 week after MTLn3 injection using the 675/30 and 720/20 nm excitation and emission filters, respectively. Monitoring of the fluorescence signals allowed us to plot growth curves for the tumours ( Fig. 4a ). For the first 2 weeks after cell injections, fluorescence brightness of the PAiRFP1- and iRFP-expressing tumours was similar, where PAiRFP2 brightness was about 4.5% of that of the iRFP tumour. After 2 weeks, brightness of the PAiRFP1 and PAiRFP2 tumours was approximately 40% and 8% of the iRFP tumour, respectively. 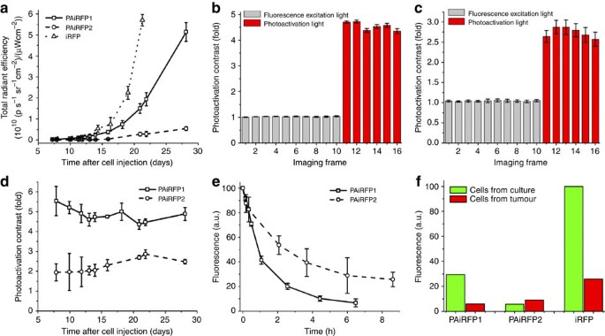Figure 4: Properties of PAiRFP1 and PAiRFP2 in mouse tumour model. (a) Tumour growth curves plotted based on increase of fluorescence brightness of PAiRFP1 (solid line), PAiRFP2 (dashed line) and iRFP (dotted line). Fluorescence brightness of PAiRFP1 and PAiRFP2 was measured after photoactivation with 660 nm 26 mW cm−2light. Photoactivation kinetics of the PAiRFP1- (b) and PAiRFP2- (c) expressing tumours in mice. The mice were imaged with 675/30 nm 6.4 μW cm−2excitation light (2 s exposure time per frame) before (frames 1–10; grey columns) and after repetitive 5 s irradiation with 660 nm 26 mW cm−2LED photoactivation light per each frame (frames 11–16; red columns). SeeSupplementary Figs S10 and S11for the respective images of mice. (d) Photoactivation contrast of PAiRFP1 (squares) and PAiRFP2 (circles) for different tumour sizes. (e) Kinetics of the dark reversion of PAiRFP1 (squares) and PAiRFP2 (circles) after complete photoactivation. (f) Mean fluorescence intensity of the cells isolated from PAiRFP1-, PAiRFP2- and iRFP-expressing tumours 5 weeks after injection, in comparison with the respective preclonal cell mixtures growing in culture. Fluorescence was analysed using flow cytometer with 640 nm excitation laser. Fluorescence intensities were normalized to absorbance of the respective protein at 640 nm and overlap of the fluorescence spectrum of the respective protein with the transmission of the emission filter. Error bars, s.d. (n=3). Figure 4: Properties of PAiRFP1 and PAiRFP2 in mouse tumour model. ( a ) Tumour growth curves plotted based on increase of fluorescence brightness of PAiRFP1 (solid line), PAiRFP2 (dashed line) and iRFP (dotted line). Fluorescence brightness of PAiRFP1 and PAiRFP2 was measured after photoactivation with 660 nm 26 mW cm −2 light. Photoactivation kinetics of the PAiRFP1- ( b ) and PAiRFP2- ( c ) expressing tumours in mice. The mice were imaged with 675/30 nm 6.4 μW cm −2 excitation light (2 s exposure time per frame) before (frames 1–10; grey columns) and after repetitive 5 s irradiation with 660 nm 26 mW cm −2 LED photoactivation light per each frame (frames 11–16; red columns). See Supplementary Figs S10 and S11 for the respective images of mice. ( d ) Photoactivation contrast of PAiRFP1 (squares) and PAiRFP2 (circles) for different tumour sizes. ( e ) Kinetics of the dark reversion of PAiRFP1 (squares) and PAiRFP2 (circles) after complete photoactivation. ( f ) Mean fluorescence intensity of the cells isolated from PAiRFP1-, PAiRFP2- and iRFP-expressing tumours 5 weeks after injection, in comparison with the respective preclonal cell mixtures growing in culture. Fluorescence was analysed using flow cytometer with 640 nm excitation laser. Fluorescence intensities were normalized to absorbance of the respective protein at 640 nm and overlap of the fluorescence spectrum of the respective protein with the transmission of the emission filter. Error bars, s.d. ( n= 3). Full size image To establish optimal conditions for complete photoactivation of PAiRFPs in vivo , we measured photoactivation kinetics of a tumour under illumination used for fluorescence read out and light irradiation used for photoactivation. Light at 675/30 nm with 6.4 μW cm −2 power used for fluorescence excitation in the IVIS Spectrum did not photoactivate PAiRFPs, allowing prolonged imaging of a non-photoactivated tumour ( Fig. 4b , imaging frames 1–10; Supplementary Figs S10 and S11 ). Here and below, the light powers are indicated on the samples. However, 5 s illumination with 660 nm light of 26 mW cm −2 led to almost complete photoactivation of the whole tumour ( Fig. 4b , imaging frames 11–16). For complete in vivo photoactivation, we further used 10 s illumination with 660 nm light of 26 mW cm −2 . The photoactivation contrast of PAiRFPs measured during development of the tumours showed no significant dependence on their size and total brightness ( Fig. 4d ). The values of photoactivation contrast were in the range of 4.4±0.3–5.5±0.7 for PAiRFP1 and 1.9±0.4–2.9±0.2 for PAiRFP2. After photoactivation, fluorescence of PAiRFP1 and PAiRFP2 in tumours decreased with the half-times of 55 and 155 min, respectively ( Fig. 4e ). Post-mortem flowcytometry analysis of PAiRFP1- and iRFP-expressing tumour cells demonstrated a similar ratio between negative and fluorescent cells (~6.1% and ~6.6% positive cells for PAiRFP1 and iRFP, respectively) that resembles the previously reported results for iRFP [20] . Mean fluorescence intensities of the PAiRFP1 and iRFP positive cells were 20% and 26%, respectively, relative to respective preclonal MTLn3 mixtures growing in culture ( Fig. 4f ). In the case of PAiRFP2, the ratio between negative and fluorescent cells isolated from a tumour was 0.72%. Interestingly, mean fluorescence intensity of the PAiRFP2 cells from the tumour was 1.6-fold higher than preclonal mixed MTLn3 cells growing in culture. Overall, in vivo data suggested that PAiRFPs are suitable for long-term expression in mammals. The ability to easily change the PAiRFPs fluorescence signal from the relaxed state to the fluorescent state by photoactivation enables simple image processing, which results in a substantially enhanced fluorescence contrast. To estimate contrast enhancement, we performed in vivo imaging of mice bearing PAiRFPs and control iRFP-expressing tumours at early stages of approximately 10 days after the MTLn3 cell injection. Subtracting images captured before photoactivation from the images captured after photoactivation resulted in the 18- and 26-fold increase in the signal-to-background ratios for the PAiRFP1 and PAiRFP2 tumours, respectively, relative to the respective unprocessed images ( Fig. 5a ). Similar procedure is not possible for permanently fluorescent iRFP because its fluorescence signal remains constant ( Fig. 5b ). Therefore, the signal-to-background ratio values for PAiRFP1 and PAiRFP2 images after this contrast enhancement procedure were 6.5- and 2.1-fold higher than that for iRFP ( Fig. 5c ). 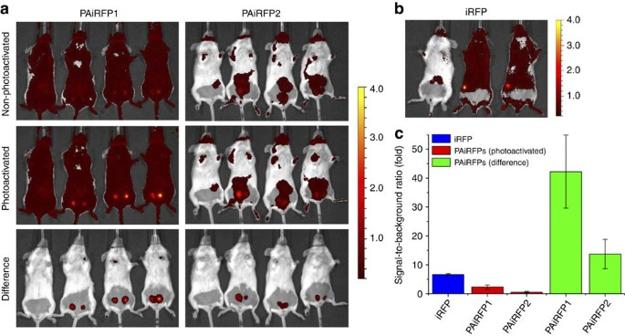Figure 5: Contrast enhancement ofin vivoimaging using PAiRFP1 and PAiRFP2. (a) Overlay of the representative light and fluorescent images of a control mouse (left on each image) and the mice bearing a 10-day old PAiRFP1-expressing tumour (left column) and a 13-day old PAiRFP2-expressing tumour (right column) before (upper row) and after photoactivation (middle row), Overlay of the representative light and fluorescent images obtained by subtracting of the ‘non-photoactivated’ image from the ‘photoactivated’ is shown in the lower row. The colour bar indicates the fluorescence radiant efficiency, multiplied by 108. (b) Overlay of the representative light and fluorescent images of a control mice (left) and the mice bearing a 10-day old iRFP-expressing tumour. The colour bar indicates the fluorescence radiant efficiency, multiplied by 108. (c) The signal-to-background ratio values calculated for the respective images inaandb. Error bars, s.d. (n=6). Figure 5: Contrast enhancement of in vivo imaging using PAiRFP1 and PAiRFP2. ( a ) Overlay of the representative light and fluorescent images of a control mouse (left on each image) and the mice bearing a 10-day old PAiRFP1-expressing tumour (left column) and a 13-day old PAiRFP2-expressing tumour (right column) before (upper row) and after photoactivation (middle row), Overlay of the representative light and fluorescent images obtained by subtracting of the ‘non-photoactivated’ image from the ‘photoactivated’ is shown in the lower row. The colour bar indicates the fluorescence radiant efficiency, multiplied by 10 8 . ( b ) Overlay of the representative light and fluorescent images of a control mice (left) and the mice bearing a 10-day old iRFP-expressing tumour. The colour bar indicates the fluorescence radiant efficiency, multiplied by 10 8 . ( c ) The signal-to-background ratio values calculated for the respective images in a and b . Error bars, s.d. ( n= 6). Full size image Selective photoactivation of PAiRFPs in vivo Low light intensity required to photoactivate PAiRFPs prompted us to perform spatially selective photoactivation within an organ in a mouse. We built a setup capable of delivering a focused beam of light of specific power to small areas of a tumour. The setup consisted of a 660 nm laser diode, a focusing lens, a mechanical shutter, a patch cable and a fibre optic cannula. We tested two methods of the selective photoactivation, dubbed ‘via skin’ and ‘via needle’ ( Fig. 6a ). 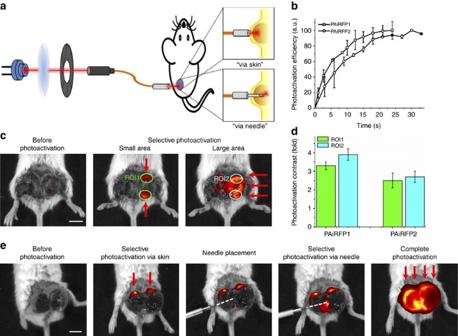Figure 6: Selective photoactivation of PAiRFP1 and PAiRFP2 in mouse tumour model. (a) Scheme of an optical device consisting of a 660 nm laser diode, a focusing lens, a mechanical shutter, a patch cable and a fibre optic cannula. Device is used for ‘via skin’ and ‘via needle’ selective photoactivation of the PAiRFP1- and PAiRFP2-expressing tumours in living mice. (b) Kinetics of via skin selective photoactivation of the PAiRFP1- (square) and PAiRFP2- (circle) expressing tumours with 660 nm laser beam of 1.5 mW total power. Photoactivation efficiency was calculated as (ROIt−ROI0)/ROImax× 100, where ROIt, ROI0and ROImaxwere total radiant efficiencies of the respective areas aftertseconds of illumination, before illumination and after complete photoactivation, respectively. (c) Overlay of the representative light and fluorescence images of a mouse bearing a 4-week old MTLn3 tumour expressing PAiRFP1 before photoactivation (left image), after selective photoactivation of two small areas (middle image) and after complete photoactivation of the whole tumour (right image). Red arrows indicate areas where the light beam was applied. (d) Average photoactivation contrast of the PAiRFP1- and PAiRFP2-expressing tumours in ROI1 and ROI2, represented onFig. 4c. Average photoactivation contrast values were obtained from 9 and 4 ROIs of PAiRFP1 and PAiRFP2 tumours, respectively. (e) Overlay of the representative light and fluorescent images of a mouse bearing a 5-week old MTLn3 tumour expressing PAiRFP2 before photoactivation (first image), after selective via skin photoactivation of two small areas (second image), with subsequent placement of the needle into the tumour (third image), selective photoactivation via needle (fourth image) and complete photoactivation of the tumours (fifth image). Red arrows indicate areas photoactivated via skin. White dashed line indicates path of the needle inside of the tumour. Error bars, s.d. (n=3). Scale bars, 1 cm. Figure 6: Selective photoactivation of PAiRFP1 and PAiRFP2 in mouse tumour model. ( a ) Scheme of an optical device consisting of a 660 nm laser diode, a focusing lens, a mechanical shutter, a patch cable and a fibre optic cannula. Device is used for ‘via skin’ and ‘via needle’ selective photoactivation of the PAiRFP1- and PAiRFP2-expressing tumours in living mice. ( b ) Kinetics of via skin selective photoactivation of the PAiRFP1- (square) and PAiRFP2- (circle) expressing tumours with 660 nm laser beam of 1.5 mW total power. Photoactivation efficiency was calculated as (ROI t −ROI 0 )/ROI max × 100, where ROI t , ROI 0 and ROI max were total radiant efficiencies of the respective areas after t seconds of illumination, before illumination and after complete photoactivation, respectively. ( c ) Overlay of the representative light and fluorescence images of a mouse bearing a 4-week old MTLn3 tumour expressing PAiRFP1 before photoactivation (left image), after selective photoactivation of two small areas (middle image) and after complete photoactivation of the whole tumour (right image). Red arrows indicate areas where the light beam was applied. ( d ) Average photoactivation contrast of the PAiRFP1- and PAiRFP2-expressing tumours in ROI1 and ROI2, represented on Fig. 4c . Average photoactivation contrast values were obtained from 9 and 4 ROIs of PAiRFP1 and PAiRFP2 tumours, respectively. ( e ) Overlay of the representative light and fluorescent images of a mouse bearing a 5-week old MTLn3 tumour expressing PAiRFP2 before photoactivation (first image), after selective via skin photoactivation of two small areas (second image), with subsequent placement of the needle into the tumour (third image), selective photoactivation via needle (fourth image) and complete photoactivation of the tumours (fifth image). Red arrows indicate areas photoactivated via skin. White dashed line indicates path of the needle inside of the tumour. Error bars, s.d. ( n= 3). Scale bars, 1 cm. Full size image For determining optimal photoactivation conditions, we initially measured kinetics of the ‘via skin’ photoactivation, which were used for all further experiments ( Fig. 6b ). Total light power at the exit of the patch cable was ~1.5 mW. Half-times of selective photoactivation of PAiRFP1 and PAiRFP2 in tumours were 4.1±0.4 and 7±2 s, respectively. We photoactivated two spots within the same tumour, with an average photoactivation contrast in the selected regions of interest (ROIs) of 3.3±0.2- and 2.5±0.4-fold for PAiRFP1- and PAiRFP2-expressing tumours, respectively (ROI1 in Fig. 6c ). After photoactivation of the whole tumour, average contrast in the selected ROIs was 3.9±0.3- and 2.7±0.3-fold for PAiRFP1 and PAiRFP2, respectively (ROI2 in Fig. 6c ). For ‘via needle’ photoactivation, a light fibre was protected with a syringe needle for its insertion into a tissue. To test this method of photoactivation, two spots in the PAiRFP2-expressing tumour were photoactivated via skin, as described above. Subsequently, the needle with the optical fibre was inserted into the middle of the tumour, and illumination was applied for 5–6 s ( Fig. 6e ). Total light power at the exit of the needle was ~0.5–1.0 mW. The fibre optic cannula with the needle inserted in the tissue can be easily disconnected from the optical setup, and the animal can be imaged. After imaging, the cannula is connected back to the device, allowing further illumination of the same spot to achieve a desirable level of photoactivation. Combining the ‘via skin’ and ‘via needle’ light irradiation techniques allowed rapid and selective photoactivation of several spots in the tumour tissue. We employed molecular evolution of a bathy BphP named At BphP2 for the purpose of developing dark-to-NIR PA FPs. As a result, we have found two variants, named PAiRFP1 and PAiRFP2, with distinctive biochemical characteristics ( Table 1 and Fig. 1 ). We have introduced 15 and 24 amino acid substitutions into AtPCD to engineer PAiRFP1 and PAiRPF2, respectively. Spectral and photochemical properties of light-active proteins are mainly determined by interactions between the chromophore and its immediate environment. We proposed the possible effects of the newly introduced amino acid residues in close proximity to the chromophore in PAiRFPs through analysis of the spectral and biochemical properties of the AtPCD variants, as well as mutagenesis and structural data available for other BphPs. We aligned the amino acid sequence of the At BphP2 PCD with the bathy BphP Pa BphP sequence from Pseudomonas aeruginosa [34] , which share 37% sequence identity ( Supplementary Fig. S12 ), to suggest the possible location of the introduced mutations in the PAiRFP tertiary structures. Next, the available crystal structures of Pa BphP-PCD in its dark-adapted Pfr state and the Pr state were used to locate the residue of interest [11] , [36] . Analysis of the alignment revealed that 12 out of 15 substitutions of PAiRPF1 reside in the GAF domain, with the remaining 3 in the PHY domain. PAiRFP2 contains 3 mutations in the PAS domain, 11 in the GAF domain and 10 in the PHY domain. In addition, according to the alignment, only three mutations (M163L, V244F and A276V) of PAiRFP1 and four mutations (M163L, S243N, V244F and A276V) of PAiRFP2 reside in the chromophore-binding pocket ( Supplementary Fig. S12 ). In Supplementary Note 1 , we proposed possible effects of the M163L, V244F and A276V mutations on the PAiRFPs photophysical and photochemical properties based on the properties of other bacteriophytochromes, such as Dr BphP, Pa BphP and their mutants, and mutants generated during molecular evolution of AtPCD. To determine the roles of all other introduced mutations, further structural, spectroscopic and mutational analysis of PAiRFPs is required. Overall, we conclude that the novel mutations in the PAiRFPs are mainly responsible for (i) altering sensitivity to ‘red’ versus ‘far-red’ light, (ii) disabling the Pr→Pfr photoconversion, (iii) decreasing dark reversion rates, (iv) increasing the extinction coefficient and quantum yield of the Pr state and (v) increasing the photoactivation contrast. The introduced mutations did not cause substantial shift of the absorbance and fluorescence spectra: parental AtPCD and its variants exhibit the similar absorbance and fluorescence maxima ( Supplementary Table S1 ). In the relaxed and photoactivated states, PAiRFP1 has absorbance maxima at 756 and 692 nm, respectively; hence, the relaxed and photoactivated states of PAiRFP1 correspond to the Pfr and Pr states, respectively. In the relaxed state, PAiRFPs exhibit residual fluorescence, which is blue-shifted relative to the photoactivated state ( Table 1 ). This fluorescence can arise from a state other than Pr, which probably exists in a thermal equilibrium with the Pfr state. Interestingly, the excitation maximum of this state corresponds to the 660-nm local maximum of the spectral dependence of photoactivation for PAiRFPs ( Table 1 and Fig. 1e ). Possibly, illumination of this state with 660 nm light can result in the formation of Pr and is an intermediate in the Pfr→Pr photoconversion pathway. We utilized low-temperature ultraviolet-visible spectroscopy to study mechanism of PAiRFPs photoconversion. To identify the intermediates involved in the PAiRFPs photocycle, we compared the calculated difference spectra for PAiRFPs photoconversion ( Fig. 2 ) with the ones available for wild-type phytochromes [14] , [15] , [16] , [17] , [18] (see Supplementary Note 2 ). These suggest that photoconversion of PAiRFPs proceeds via intermediates similar to that of wild-type phytochromes, which, we believe, are involved in the alternation of BV conformations and re-arrangement of protein moieties around BV ( Fig. 2i ). Thus, photoactivation of PAiRFPs does not seem to involve chemical modifications of the BV chromophore except its protonation–deprotonation and isomerization. Although PAiRFPs in mammalian cells are less bright than iRFP, their brightness is sufficient for imaging cells in culture and in live mice. The noticeable difference in PAiRFP brightness in vitro and in mammalian cells can be possible explained by a lower affinity to BV and/or instability of PAiRFP holoproteins, as it has been suggested for IFP1.4 (ref. 21 ). However, imaging with PAiRFPs does not require BV administration, as endogenous BV in mammalian cells is sufficient for formation of the fluorescent apoprotein. Using the xenograft tumour mouse model, we showed applicability of PAiRFPs for whole-body imaging. Tumour growth dynamics and post-mortem analysis of tumour cells expressing PAiRFPs suggest that the proteins are suitable for long-term expression in mammals. In addition, photoactivation of PAiRFPs is rapid, easy and allows simultaneous tissue photolabelling in several mice using an LED array. The described ‘via skin’ and ‘via needle’ photoactivation setups allow precise and gradual photoactivation of a selected ROI. Photoactivation contrast does not depend on the size and brightness of the expressing tissue, making PAiRFPs reliable probes for semi-quantitative in vivo imaging. The ability to change the PAiRFP fluorescence signal by photoactivation has allowed to substantially increase the signal-to-background ratio values of the in vivo images, thus resulting in an order of magnitude of higher fluorescence contrast ( Fig. 5 ). Although the PAiRFP2-expressing tumour was about 10-fold less bright after photoactivation than the iRFP-expressing tumour, the processed signal-to-background ratio for PAiRFP2 was more than twice higher than for iRFP. The possibility to subtract the PAiRFPs images before and after photoactivation makes these proteins advantageous over permanently fluorescent NIR FPs for imaging in vivo when there are typically high autofluorescence levels. This approach is particularly important for imaging of small organs and tissues such as early tumours, which provide low fluorescence signals due to the small number of fluorescent cells. Potentially, multiple photoactivation—dark relaxation cycles of PAiRFPs may be useful to allow unambiguous assignment of the signals to PAiRFPs and to improve spatial resolution of in vivo imaging. PAiRFPs extend the set of available and widely used PA FPs derived from GFP-like proteins [28] , [37] . However, PAiRFPs possess several features distinct of the GFP-like PA FPs. First, both excitation and emission fluorescence spectra of PAiRFPs lie within the NIR ‘optical window’ and are >50 nm red-shifted relative to the most red-shifted photoswitchable GFP-like protein, PSmOrange [38] . Second, PAiRFPs are photoactivated by NIR light, whereas the most of the GFP-like PA FPs are activated by ultraviolet light, with the exception of a few reversibly photoswitchable RFPs, which are photoconverted by orange light [39] . Third, the light power required for PAiRFP photoactivation is orders of magnitude lower than that required for GFP-like PA FP photoactivation ( Supplementary Table S2 ). For comparison, the photoconversion energy density required for the PSmOrange [38] and PATagRFP [40] photoconversion is ~5,000-fold higher than that for PAiRFPs. The latter can be explained by the distinct molecular mechanisms of chromophore transformations involved in photoactivation. Phototransformation of phytochromes and their derivatives only involves isomerization and protonation–deprotonation of the chromophore [4] , [5] , whereas photoconversion of GFP-like FPs involve chemical modification of the chromophores, which requires higher activation energy [37] , [41] . PAiRFPs can be completely photoactivated in vivo within seconds, whereas in vivo photoactivation of PSmOrange takes more than a half of hour [38] . Lastly, in vivo photoactivation of PAiRFPs does not require sophisticated equipment, in contrast to, for example, Dendra PA FP photoactivation [42] . These features make PAiRFPs advantageous over the GFP-like PA FPs for in vivo photolabelling and imaging cells, tissues and whole mammals. Mutagenesis and screening of the libraries An At BphP2 gene was kindly provided by Eric Giraud. A PCR-amplified Bgl II– Asu II fragment encoding AtPCD (first 502 amino acids of the At BphP2 protein with the insertion of the MAGLEYK sequence on the C-terminus) was cloned into the pBAD/His-B vector (Invitrogen). Random mutagenesis was performed with GeneMorph II Random Mutagenesis Kit (Stratagene) using conditions resulting in a mutation frequency up to 16 mutations per 1,000 bp. After mutagenesis, a mixture of the mutants was electroporated into LMG194 host cells (Invitrogen) containing the pWA23h plasmid, which facilitates biliverdin synthesis. The pWA23h plasmid contained the rhamnose promoter from the pWA21 plasmid [43] , Kan resistance and COLA origin parts from a pCOLADuet-1 plasmid (Novagen). First, the Avr II/ Pci I fragment containing Kan resistance and COLA origin was PCR amplified from pCOLADuet-1 plasmid and inserted into a pWA21h- Avr II/ Not I vector. Then, a hmuO gene encoding Bradyrhizobium ORS278 haem oxygenase was PCR amplified from pBAD/His-B-RpBphP2-hmuO plasmid [44] and swapped with the EGFP gene in the pWA21- Avr II/ Not I plasmid. Typical mutant libraries consisted of about 10 6 –10 8 independent clones. The LMG194 cells were grown at 37 °C in RM minimal medium supplemented with ampicillin, kanamycin and 100 μM of 5-aminolevulinic acid (ALA). Protein expression in the libraries was induced with 0.002% arabinose and 0.02% rhamnose. The cells were grown up to 18 h at 37 °C. Before FACS screening, bacterial cells were washed with PBS containing 1 mM EDTA and then diluted with PBS to optical density of 0.02 at 600 nm. Cell suspensions were activated using a 750 nm 60 mW cm −2 LED array (20 nm of emission half-width and 1.7 cm diameter of light-emitting zone (Marubeni)) or a 660 nm 26 mW cm −2 LED array (20 nm of emission half-width and 17 cm diameter of light-emitting zone (90 W UFO LED; Grow Light)). The library photoactivation consisted of ~5 min illumination of the bacterial suspension mixed on ice. After photoactivation, the libraries were screened using MoFlo XDP (Beckman Coulter) FACS equipped with Argon, Krypton and Argon–Krypton mixed-gas lasers. Typically about 10 sizes of each library were sorted using 647 nm excitation line and 680 nm LP emission filter (Chroma). The brightest collected near-infrared bacterial cells were recovered in SOC medium at 37 °C for 1 h, then grown on LB/ampicillin/kanamycin petri dishes supplemented with 0.02% arabinose, 0.2% rhamnose, 100 μM ALA and 50 μM FeCl 3 overnight at 37 °C followed by incubation at 4 °C. The dishes were analysed with Leica MZ16F fluorescence stereomicroscope equipped with the 650/45 nm excitation and 690 nm LP emission filters (Chroma) and a CCD (charge-coupled device) camera before and after photoactivation with 750 or 660 nm light for 5–30 s. Approximately 20–50 of the brightest NIR clones, having the highest contrast after photoactivation, with minimal rate of dark reversion were selected, and their DNA was sequenced. A mixture of several selected mutants was then used as a template for the next round of mutagenesis. Protein characterization in vitro The At BphP2 mutants and iRFP with polyhistidine tags on the N-terminus were expressed in LMG194 bacterial cells grown in RM medium supplemented with ampicillin, kanamycin, 0.002% arabinose, 0.02% rhamnose and 100 μM ALA for 15–18 h at 37 °C and then for 24 h at 18 °C. Proteins were purified using Ni-NTA agarose (Qiagen) according to the manufacturer’s protocol with minor modification. In wash buffer, 400 mM imidazole was substituted with 100 mM EDTA. For spectroscopy, photoactivation of purified proteins was performed with 750 or 660 nm light in 50 μl quartz microcuvette (Starna Cells) at room temperature in PBS. Low-temperature ultraviolet-visible absorption spectra were measured in PBS. The fluorescence spectra and spectral dependence of the maximal photoactivation rate were measured using a FluoroMax-3 spectrofluorometer (Jobin Yvon). Fluorescence spectra of the relaxed PAiRFPs were measured using plate reader SpectraMax-M2 (Molecular Devices). For absorbance measurements, a Hitachi U-2000 spectrophotometer was used. Background light scattering was removed by subtracting a fitted λ 4 curve from the measured spectrum. To determine extinction coefficients, we used a direct measurement of protein concentrations with a BCA protein assay kit (Pierce), followed by the calculation of extinction coefficients using a Beer–Lambert–Bouguer equation. For determination of quantum yield, fluorescence signal of purified proteins was compared with that of the equally absorbing iRFP [20] . pH titrations were done using a series of buffers (100 mM sodium acetate, 300 mM NaCl for pH 2.5–5.0 and 100 mM NaH 2 PO 4 , 300 mM NaCl for pH 4.5–9.0). Mammalian plasmids and cell culture To construct pPAiRFP1-N1 and pPAiRFP2-N1 plasmids, the respective genes were PCR amplified as Bgl II– Not I fragments and swapped with the EGFP gene in pEGFP-N1 (Clontech). The pDualCMV-PAiRFP1-EGFP, pDualCMV-PAiRFP2-EGFP and pDualCMV-iRFP-EGFP plasmids for co-expression of non-targeted PAiRFPs and iRFP with EGFP were constructed by insertion of the Afl II– Afl II fragment containing CMV promoter and EGFP gene into the pPAiRFPs-N1 and piRFP-N1 vectors, digested by Afl II and dephosphorylated. Met-1 and HeLa cell lines were grown in DMEM containing 10% FBS, penicillin–streptomycin and 2 mM glutamine (Invitrogen). Cells were cultured in 35-mm glass bottom culture dishes with no. 1 cover glasses (MatTek). MTLn3 rat adenocarcinoma cells were cultured in αMEM (Life Technologies) with 5% FBS and 0.5% penicillin–streptomycin (Life Technologies). Plasmid transfections were performed using an Effectene reagent (Qiagen) according to the manufacturer’s protocol. Establishing cell lines and orthotopic injection in mammary glands were performed as previously described [45] . Imaging of HeLa cells was performed 48 h after transfection. HeLa cells were imaged using an Olympus IX81 inverted epifluorescence microscope equipped with a 200 W metal-halide arc lamp (Lumen220Pro, standardly equipped with 800 nm cold mirror; Prior), a × 60 1.35 numerical aperture oil immersion objective lens (UPlanSApo; Olympus) and standard Cy5.5 filter set (665/45 nm exciter and 725/50 nm emitter) (Chroma). Photobleaching experiments were performed in Met-1 mammalian cells stably expressing PAiRFP variants using an Olympus IX81 inverted epifluorescence microscope equipped with the 200 W metal-halide arc lamp (Prior), a × 60 1.35 numerical aperture oil immersion objective lens (UPlanSApo; Olympus), and standard Cy5.5 filter set (Chroma). Raw data were normalized to the absorbance spectra and extinction coefficients of the proteins, the spectrum of the 200 W arc lamp and transmission of the 665/45 nm photobleaching filter. In vivo fluorescence imaging One million MTLn3 cells stably expressing PAiRFP1, PAiRFP2 or iRFP alone were injected into the mammary gland of SCID/NCr mice (female, 5–7 weeks old) (Taconic) and imaged starting 1 week later using an IVIS Spectrum instrument (PerkinElmer) in epifluorescence mode. The IVIS Spectrum was equipped with the 675/30 and 720/20 nm excitation and emission filters for PAiRFPs and iRFP imaging. Belly fur was removed using a depilatory cream. Mice were fed with AIN-93M Maintenance Purified Diet (TestDiet) to reduce intrinsic autofluorescence level. Before imaging, mice were kept in the darkness for 8–10 h. Complete photoactivation of tumours was performed with the 660 nm 26 mW cm −2 LED array (90 W UFO LED; Grow Light). The LED array allowed for simultaneous evenly distributed illumination of up to five mice on the IVIS Spectrum stage. For spatially selective photoactivation, the optical setup shown in Fig. 6a was used. The 660 nm laser diode (120 mW), fibre optic cannula (200 and 400 μm core) and optogenetic patch cable (200 and 400 μm core, 50 cm long) were from Thorlabs. Total light power used for ‘via skin’ and ‘via needle’ photoactivation was ~1.5 and ~0.5–1.0 mW, respectively. The PAiRFP- and iRFP-expressing MTLn3 tumours were excised postmortem, chopped into pieces, washed with PBS supplemented with 2% of bovine serum albumin and subsequently filtered through sieves and a 35 μm filter. FACS analysis was perform with the LSRII cytometer (BD Biosciences) equipped with a 640-nm laser and a 730/45 nm emission filter. All animal experiments were performed in an AAALAC-approved facility using protocols approved by the Albert Einstein College of Medicine Animal Usage Committee. Accession codes. Nucleotide sequences for PAiRFP1 and PAiRFP2 have been deposited in NCBI GenBank Nucleotide database under accession codes KF006822 and KF006823 , respectively. How to cite this article : Piatkevich, K.D. et al. Far-red light photoactivatable near-infrared fluorescent proteins engineered from a bacterial phytochrome. Nat. Commun. 4:2153 doi: 10.1038/ncomms3153 (2013)